Stabilization and targeting of INO80 to replication forks by BAP1 during normal DNA synthesis The INO80 chromatin-remodelling complex has been implicated in DNA replication during stress in yeast. However, its role in normal DNA replication and its underlying mechanisms remain unclear. Here, we show that INO80 binds to replication forks and promotes fork progression in human cells under unperturbed, normal conditions. We find that Ino80 , which encodes the catalytic ATPase of INO80, is essential for mouse embryonic DNA replication and development. Ino80 is recruited to replication forks through interaction with ubiquitinated H2A—aided by BRCA1-associated protein-1 (BAP1), a tumour suppressor and nuclear de-ubiquitinating enzyme that also functions to stabilize Ino80. Importantly, Ino80 is downregulated in BAP1-defective cancer cells due to the lack of an Ino80 stabilization mechanism via BAP1. Our results establish a role for INO80 in normal DNA replication and uncover a mechanism by which this remodeler is targeted to replication forks, suggesting a molecular basis for the tumour-suppressing function of BAP1. The eukaryotic cell genome is compacted into chromatin containing nucleosomes as repeating structural units, each of which consists of a DNA segment wrapped around the histone octamer. As the nucleosome inhibits protein access to its DNA, mechanisms are necessary to address this fundamental barrier to the chromosomal processes in the nucleus, such as DNA replication. For instance, nucleosomes must be reconfigured or disassembled ahead of the fork for DNA polymerase to proceed during replication elongation. In addition, nucleosomes need to be reassembled behind the fork to restore pre-replication chromatin and its epigenetic state. Dysfunction and/or deregulation in such chromatin control can promote perturbation of DNA synthesis and, consequently, DNA damage, which can potentially lead to genome instability and the development of diseases such as cancer [1] , [2] . ATP-dependent chromatin remodelling is the key mechanism for chromatin alteration. INO80 is the evolutionarily conserved SWI/SNF family chromatin-remodelling complex, which consists of at least 15 subunits, including the Ino80 ATPase, and can alter chromatin structure by nucleosome sliding, histone eviction and histone exchange [3] , [4] . In addition to transcription, INO80 is involved in various chromosomal processes, including DNA repair, telomere regulation, centromere stability and chromosome segregation [5] , [6] . Furthermore, recent studies have implicated INO80 in DNA replication. In yeast, INO80 functions in the stabilization and restarting of stalled forks induced by replication stresses, such as nucleotide depletion by hydroxyurea (HU) treatment [7] , [8] , [9] . A study has suggested that INO80 functions in normal DNA replication in human cells [10] . Consistent with its role in various chromosomal processes, INO80 is critical for the maintenance of genome stability [10] , [11] , [12] , [13] . BRCA1-associated protein-1 (BAP1) is a nuclear de-ubiquitinating enzyme that contains the ubiquitin carboxy (C)-terminal hydrolase domain [14] . Earlier studies have shown that BAP1 is deleted or mutated in various human cancer cell lines and that re-expression of BAP1 in H226 human non-small cell lung cancer (or mesothelioma) cells lacking BAP1 reverses their tumorigenicity [14] , [15] , [16] . Importantly, a series of recent studies has identified inactivating mutations of BAP1 in various human cancers with high frequency in pleural malignant mesothelioma (MPM), uveal melanoma and cutaneous melanoma, indicating that germline BAP1 mutations cause the tumorigenesis of these cancers [17] , [18] , [19] , [20] , [21] , [22] , [23] . A recent study reported that BAP1 disruption in mice leads to the development of myeloid neoplasia [24] . These studies have established BAP1 as a bona fide tumour suppressor. BAP1 has been shown to function in various cellular processes, including transcription, cell cycle and proliferation, cell death, cellular differentiation, glucose metabolism and the DNA damage response [25] . Many important issues regarding the function of INO80 in DNA replication have remained unsolved. Although yeast INO80 functions in the stabilization and restarting of stress-induced stalled forks, its role in normal DNA replication remains unclear, with inconsistent results provided by different research groups [7] , [8] , [9] . To add complexity, a study reported that yeast INO80 has a specific role in DNA damage tolerance rather than replication fork progression or stability [26] . A study of the human INO80 did not provide evidence for direct involvement in DNA replication [10] . Therefore, further studies are necessary to clearly define the role of INO80 in DNA replication under normal and stressed conditions. In addition, the mechanisms that regulate INO80 function in replication, particularly how it is targeted to replication forks, are unknown. Here, we demonstrate direct involvement of INO80 in replication fork progression during normal DNA synthesis and report a novel mechanism by which BAP1 stabilizes and targets INO80 to replication forks. Importantly, we provide evidence suggesting that inactivating mutations of BAP1 can cause Ino80 downregulation during tumorigenesis. Direct role of INO80 in normal replication fork progression Because our earlier study used cytological methods to show that Ino80 formed nuclear foci overlapping with proliferating cell nuclear antigen (PCNA), a protein specifically associated with replication forks, whether Ino80 directly participates in DNA replication is unknown. To address this issue, we labelled DNA of cells under normal culture conditions with ethynyl deoxyuridine (EdU) to detect proteins associated with replicating DNA in the form of extended, intact chromatin by immunofluorescence microscopy [27] . As expected, PCNA colocalized with the EdU-labelled chromatin ( Fig. 1a , top panel), validating the assay. Notably, Ino80 colocalized with the EdU-labelled chromatin fibres ( Fig. 1a , middle panel) and overlapped with PCNA (bottom panel), indicating that INO80 binds to replication forks. INO80 appears to associate with a majority of replication forks in a given time as almost all of the EdU-labelled chromatin fibres that were detected overlapped with Ino80. INO80 binding to replication forks was also demonstrated using a different approach (see below). 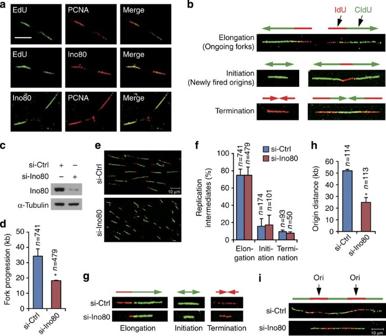Figure 1: Direct role of INO80 in replication fork progression during normal DNA synthesis. (a) Chromatin fibre assay. EdU-labelled, extended chromatin fibres were dually stained for EdU and PCNA (top panel) or EdU and Ino80 (middle panel). Extended chromatin fibres with no EdU labelling were dually stained for Ino80 and PCNA (bottom panel). Scale bar, 10 μm. (b) Confocal images of the IdU/CldU-labelled DNA fibres representing the various replication intermediates were captured in the experiments described inc–e. (c) Immunoblot for siRNA knockdown of Ino80 in HeLa cells. (d) DNA fibre assay. Average track lengths of IdU and CldU incorporation were converted to base pairs and graphed (n=3). (e) Representative confocal images ford. (f) The frequency of various replication intermediates inc–ewas graphed (n=3). (g) Representative confocal images forf. (h) Average distance of the replication origin inc–ewas graphed (n=3). (i) Representative confocal images forh. *P<0.001;n, average number of counted fibres; error bars, mean±s.e.m. Figure 1: Direct role of INO80 in replication fork progression during normal DNA synthesis. ( a ) Chromatin fibre assay. EdU-labelled, extended chromatin fibres were dually stained for EdU and PCNA (top panel) or EdU and Ino80 (middle panel). Extended chromatin fibres with no EdU labelling were dually stained for Ino80 and PCNA (bottom panel). Scale bar, 10 μm. ( b ) Confocal images of the IdU/CldU-labelled DNA fibres representing the various replication intermediates were captured in the experiments described in c – e . ( c ) Immunoblot for siRNA knockdown of Ino80 in HeLa cells. ( d ) DNA fibre assay. Average track lengths of IdU and CldU incorporation were converted to base pairs and graphed ( n =3). ( e ) Representative confocal images for d . ( f ) The frequency of various replication intermediates in c – e was graphed ( n =3). ( g ) Representative confocal images for f . ( h ) Average distance of the replication origin in c – e was graphed ( n =3). ( i ) Representative confocal images for h . * P <0.001; n , average number of counted fibres; error bars, mean±s.e.m. Full size image To evaluate the impact of INO80 on normal DNA replication and determine the steps of the replication cycle in which INO80 functions, we labelled DNA of normally growing cells consecutively with iodo-deoxyuridine (IdU) and chloro-deoxyuridine (CldU) and detected de novo DNA synthesis at the level of individual DNA molecules by extending and visualizing the labelled DNA by immunofluorescence microscopy. Thus, we could measure the replication rate and distinguish the different replication intermediates representing elongation, initiation or termination ( Fig. 1b ) [28] . Depleting Ino80 from the cells using specific small interfering RNA (siRNA; Fig. 1c ) largely decreased the track length of IdU/CldU incorporation ( Fig. 1d,e ) without affecting the frequency of various replication intermediates ( Fig. 1f,g ), indicating that INO80 promotes fork progression rather than regulating replication initiation or termination. Consistent with these results, the Ino80-deficient cells exhibited a much shorter origin distance than the control cells ( Fig. 1h,i ), compensating for slow replication. These results are consistent with our previous observations that Ino80-deficient cells are normal in entering S phase but defective in traversing it [10] . Taken together, our data show that INO80 has a direct role in fork progression during normal DNA replication. Ino80 is essential for mouse embryonic DNA replication To investigate the in vivo function of INO80, we disrupted Ino80 in mice by replacing the first three protein-coding exons with a PGK-neomycin resistance cassette using gene targeting ( Supplementary Fig. 1a–c ). Wild-type (WT) and Ino80 +/− mice were born alive in a normal Mendelian ratio, whereas no Ino80 −/− mice were observed among 175 live births from heterozygous intercrosses ( Supplementary Fig. 1d ), indicating that the targeted disruption of Ino80 resulted in embryonic lethality. While most of the Ino80 +/− mice survived without obvious phenotypic abnormalities, approximately 13% displayed a significantly smaller body size than WT, and most of these mice died within 10 weeks after birth. However, further analysis is required to verify the significance of these haploinsufficient phenotypes. To determine when Ino80 −/− embryos die, we analysed embryos from heterozygous intercrosses at various times of gestation. At E10.5 and later points, none of the 53 embryos analysed were Ino80 −/− . A few Ino80 −/− embryos were observed at E9.5 and E8.5, but these embryos appeared to die or stop growing before E8.5 ( Supplementary Fig. 1d,e ). There were no noticeable deficits in Ino80 +/− embryos ( Supplementary Fig. 1d,e ). For further analysis of the Ino80 -null embryonic lethality, two-cell embryos were obtained from heterozygous intercrosses at E1.5 and were grown in a culture dish for 3 days ( Supplementary Fig. 1f ). All nine littermate embryos normally developed to blastocysts ( Supplementary Fig. 1g ), indicating that Ino80 disruption did not affect embryonic development to the blastocyst stage. Next, the blastocyst-stage embryos were collected from heterozygous intercrosses at E3.5 and were cultured for several days with monitoring every day ( Fig. 2a ). After 1–2 days of culture, the spherical blastocysts flattened onto the culture dish with spreading of the trophoblast cells on which the inner cell mass (ICM) grew. The ICM of two of nine littermate embryos, which were most likely Ino80 −/− , stopped proliferating and were completely lost after 4 days in culture, whereas the ICM of the remaining embryos continued to grow throughout the time course analysed. In parallel experiments, none of the seven embryos collected from WT × Ino80 +/− crosses showed defects in ICM growth ( Fig. 2b and Supplementary Fig. 1h ). These results show that Ino80 is essential for ICM proliferation during early embryogenesis. 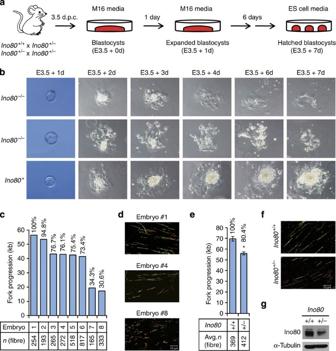Figure 2:Ino80is essential for embryonic DNA replication and development in mice. (a) Schematic procedure for thein vitroculture of mouse embryos. (b) Harvested blastocysts were photographed at the indicated times. The top two panels show two of nine embryos from theIno80+/−intercross that displayed severe ICM defects (embryos #3 and #5 inSupplementary Fig. 1h). The bottom panel shows one of the seven embryos fromIno80+/−×Ino80+/+(embryo #7 inSupplementary Fig. 1h). (c) Eight embryos obtained from theIno80+/−intercross were subjected to the DNA fibre assay. The fork progression of a most replication-proficient embryo was set as 100%, and the relative percentages of the fork progression of the remaining embryos were calculated. The number of DNA fibres that were counted for each embryo is shown. (d) Representative confocal images forc. (e) DNA fibre assay with WT andIno80+/−MEFs. The average number of counted fibres for each sample is shown.n=3; *P<0.001; error bars, mean±s.e.m. (f) Representative confocal images fore. (g) Immunoblot for the Ino80 levels in WT andIno80+/−MEFs. Figure 2: Ino80 is essential for embryonic DNA replication and development in mice. ( a ) Schematic procedure for the in vitro culture of mouse embryos. ( b ) Harvested blastocysts were photographed at the indicated times. The top two panels show two of nine embryos from the Ino80 +/ − intercross that displayed severe ICM defects (embryos #3 and #5 in Supplementary Fig. 1h ). The bottom panel shows one of the seven embryos from Ino80 +/ − × Ino80 +/+ (embryo #7 in Supplementary Fig. 1h ). ( c ) Eight embryos obtained from the Ino80 +/ − intercross were subjected to the DNA fibre assay. The fork progression of a most replication-proficient embryo was set as 100%, and the relative percentages of the fork progression of the remaining embryos were calculated. The number of DNA fibres that were counted for each embryo is shown. ( d ) Representative confocal images for c . ( e ) DNA fibre assay with WT and Ino80 +/ − MEFs. The average number of counted fibres for each sample is shown. n =3; * P <0.001; error bars, mean±s.e.m. ( f ) Representative confocal images for e . ( g ) Immunoblot for the Ino80 levels in WT and Ino80 +/ − MEFs. Full size image To determine whether Ino80 −/− embryos were defective in DNA replication, we conducted the DNA fibre assay with blastocysts cultured for 1 day after collection from Ino80 +/− intercrosses (E3.5+1d). When the eight littermate embryos were arranged in order of their replicative capacity, they could be divided into three groups: two embryos with high proficiency, four with medium proficiency (~3/4 levels of the first group) and two with low proficiency (~1/3 levels of the first group; Fig. 2c,d ). Because their ratio coincided with Mendelian law, the three groups of embryos were most likely WT, Ino80 +/− and Ino80 −/− , respectively. When we conducted two additional similar experiments, we obtained virtually the same results ( Supplementary Fig. 1i,j ). In support of our interpretation, Ino80 +/− mouse embryonic fibroblasts (MEFs) were 20% less efficient in replication than WT ( Fig. 2e–g ). The frequency of the replication intermediates was not different among the three groups of embryos ( Supplementary Fig. 1k ) or between WT and Ino80 +/− MEFs ( Supplementary Fig. 1l ). Therefore, INO80 promotes replication fork progression in mouse embryonic cells, and this INO80 function seems to be critical for early stage embryogenesis. BAP1 interacts with INO80 and forms replication foci To better understand the INO80 function in DNA replication, we conducted a yeast two-hybrid screen to identify the proteins that interact with Ino80. Among many candidates for the Ino80-interacting proteins ( Supplementary Table 1 ), we chose BAP1 for further investigation because our initial study showed that it formed distinct nuclear foci overlapping with Ino80 in S-phase cells. The interaction between BAP1 and Ino80 was verified by immunoprecipitation in various cell types, such as 293T ( Fig. 3a,b ), HCT116 ( Supplementary Fig. 2 ) and HeLa cells (see below). The mapping experiments showed that the helicase-SANT-associated (HSA) domain of Ino80 and BRCA1 interaction domain located at the C terminus of BAP1 are involved in the interaction of these two proteins ( Fig. 3c,d ). 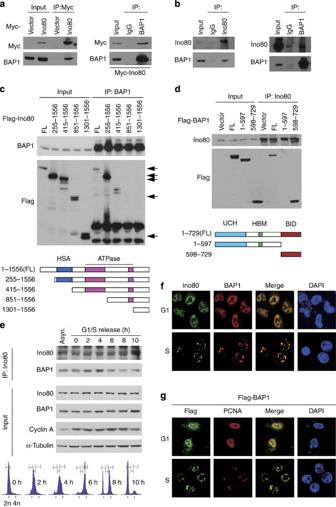Figure 3: BAP1 interacts with Ino80 and forms replication foci in S phase. (a) Myc-tagged proteins (left) or BAP1 (right) were immunoprecipitated from 293T cells expressing Myc-Ino80 and were subjected to immunoblotting. (b) Ino80 (left) or BAP1 (right) were immunoprecipitated from 293T cells and subjected to immunoblotting. (c) BAP1 was immunoprecipitated from 293T cells expressing full-length or various truncation mutants of Flag-Ino80 and were subjected to immunoblotting. (d) Ino80 was immunoprecipitated from 293T cells expressing full-length or truncation mutants of Flag-BAP1 and were subjected to immunoblotting. HBM, HCT-1-binding motif. (e) Ino80 was immunoprecipitated from HCT116 cells in normal culture (asynchronised) or at various times after release from a double thymidine block (G1/S arrest) and then were subjected to immunoblotting (top). The corresponding cell cycle profiles are shown (bottom). HeLa cells (f) and 293T cells expressing Flag-BAP1 (g) were dually stained as indicated, and the confocal images of G1- and S-phase cells were captured. Figure 3: BAP1 interacts with Ino80 and forms replication foci in S phase. ( a ) Myc-tagged proteins (left) or BAP1 (right) were immunoprecipitated from 293T cells expressing Myc-Ino80 and were subjected to immunoblotting. ( b ) Ino80 (left) or BAP1 (right) were immunoprecipitated from 293T cells and subjected to immunoblotting. ( c ) BAP1 was immunoprecipitated from 293T cells expressing full-length or various truncation mutants of Flag-Ino80 and were subjected to immunoblotting. ( d ) Ino80 was immunoprecipitated from 293T cells expressing full-length or truncation mutants of Flag-BAP1 and were subjected to immunoblotting. HBM, HCT-1-binding motif. ( e ) Ino80 was immunoprecipitated from HCT116 cells in normal culture (asynchronised) or at various times after release from a double thymidine block (G1/S arrest) and then were subjected to immunoblotting (top). The corresponding cell cycle profiles are shown (bottom). HeLa cells ( f ) and 293T cells expressing Flag-BAP1 ( g ) were dually stained as indicated, and the confocal images of G1- and S-phase cells were captured. Full size image To examine whether INO80 interacts with BAP1 specifically during S phase, we collected asynchronized cells or cells at 2-h intervals after release from G1/S arrest by double thymidine blockade for immunoprecipitation. The Ino80-BAP1 interaction was readily detected from the asynchronized cells, and this interaction was not significantly enhanced, if any, during S phase ( Fig. 3e ). In the immunohistochemistry, Ino80 and BAP1 were co-stained evenly across the nucleus, excluding nucleoli in G1, and formed distinct foci overlapping with each other in S phase ( Fig. 3f ), and the BAP1 foci overlapped with PCNA in S phase ( Fig. 3g ). The overlapping of BAP1 and Ino80 foci was sustained throughout the S phase ( Supplementary Fig. 3a ) as was the overlapping between Ino80 and PCNA foci ( Supplementary Fig. 3b ). These results show that, although the interaction between Ino80 and BAP1 occurs throughout the cell cycle, both proteins accumulate into replication foci specifically during S phase. BAP1 stabilizes Ino80 by de-ubiquitination The ubiquitin–proteasome pathway is the major molecular mechanism that regulates the concentration of particular proteins in the cells by ubiquitinating the proteins for proteasome-mediated degradation [29] . Because BAP1 is a de-ubiquitinating enzyme and interacts with Ino80, we asked whether BAP1 de-ubiquitinates and stabilizes Ino80. We observed that Ino80 could be ubiquitinated within cells ( Fig. 4a ), and its cellular levels were increased by treatment with the proteasome inhibitor MG132 ( Fig. 4b,c ), indicating that Ino80 is under the control of the ubiquitin-mediated proteasomal degradation pathway. Ectopically expressing WT BAP1, but not the C91S mutant lacking catalytic activity, in the cells reduced the Ino80 ubiquitination ( Fig. 4d ), and conversely, depleting BAP1 from the cells using specific siRNA increased Ino80 ubiquitination ( Fig. 4e ), indicating that BAP1 is responsible for Ino80 de-ubiquitination. 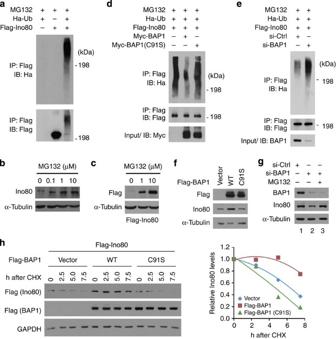Figure 4: BAP1 stabilizes Ino80 by de-ubiquitination. (a) After treatment with 10 μM MG132, Flag-tagged proteins were immunoprecipitated from 293T cells expressing Flag-Ino80 and/or Ha-tagged ubiquitin (Ha-Ub) and then were subjected to immunoblotting. After treatment with increasing concentrations of MG132, the Ino80 (b) and Flag-Ino80 levels (c) were determined by immunoblotting. (d) After treatment with MG132, Flag-tagged proteins were immunoprecipitated from the cells expressing Ha-Ub and Flag-Ino80 along with WT or C91S Myc-BAP1 and then were subjected to immunoblotting. (e) BAP1 was depleted by siRNA in the cells expressing Ha-Ub and Flag-Ino80. Flag-tagged proteins were immunoprecipitated following MG132 treatment and then were subjected to immunoblotting. (f) The effects of BAP1 overexpression on Ino80 levels. (g) The Ino80 levels in cells depleted of BAP1 were determined by immunoblotting before or after MG132 treatment. (h) (Left) After co-transfection with the indicated expression vectors, the cells were collected at various times after cycloheximide (CHX) treatment and then were subjected to immunoblotting. (Right) The relative intensities of Flag-Ino80 bands were depicted graphically after normalization to GAPDH. Similar results were obtained from four independent experiments. Figure 4: BAP1 stabilizes Ino80 by de-ubiquitination. ( a ) After treatment with 10 μM MG132, Flag-tagged proteins were immunoprecipitated from 293T cells expressing Flag-Ino80 and/or Ha-tagged ubiquitin (Ha-Ub) and then were subjected to immunoblotting. After treatment with increasing concentrations of MG132, the Ino80 ( b ) and Flag-Ino80 levels ( c ) were determined by immunoblotting. ( d ) After treatment with MG132, Flag-tagged proteins were immunoprecipitated from the cells expressing Ha-Ub and Flag-Ino80 along with WT or C91S Myc-BAP1 and then were subjected to immunoblotting. ( e ) BAP1 was depleted by siRNA in the cells expressing Ha-Ub and Flag-Ino80. Flag-tagged proteins were immunoprecipitated following MG132 treatment and then were subjected to immunoblotting. ( f ) The effects of BAP1 overexpression on Ino80 levels. ( g ) The Ino80 levels in cells depleted of BAP1 were determined by immunoblotting before or after MG132 treatment. ( h ) (Left) After co-transfection with the indicated expression vectors, the cells were collected at various times after cycloheximide (CHX) treatment and then were subjected to immunoblotting. (Right) The relative intensities of Flag-Ino80 bands were depicted graphically after normalization to GAPDH. Similar results were obtained from four independent experiments. Full size image Next, we examined whether BAP1 stabilizes Ino80. The ectopic expression of WT BAP1, but not the C91S mutant, increased Ino80 ( Fig. 4f ), and siRNA depletion of BAP1 decreased Ino80 ( Fig. 4g , lanes 1 and 2). Importantly, the Ino80 decrease by BAP1 depletion was reversed by treatment with MG132 ( Fig. 4g , lane 3), indicating that BAP1 regulates the Ino80 level via the proteasome degradation pathway. To determine whether BAP1 increases Ino80 by extending its half-life, the cellular levels of Ino80 were monitored after treatment with the translational inhibitor cycloheximide. In the absence of de novo protein synthesis, Ino80 decayed in the cells containing a control vector with a half-life of approximately 6 h. Overexpressed BAP1 extended the half-life of Ino80 far beyond 6 h. The de-ubiquitinating activity of BAP1 was necessary for Ino80 accumulation because the C91S mutant did not increase the half-life of Ino80 ( Fig. 4h ). Taken together, we concluded that BAP1 de-ubiquitinates and stabilizes Ino80 by extending its half-life. BAP1 contributes to DNA replication via Ino80 Having found that BAP1 stabilizes Ino80, we asked whether BAP1 contributes to DNA replication. Depleting BAP1 decreased Ino80 as expected and also decreased replication elongation ( Fig. 5a–c ). The replication defect by BAP1 depletion was similar in extent to that by Ino80 depletion but was not further exacerbated by the simultaneous depletion of the two proteins ( Fig. 5a–c ), suggesting that BAP1 and INO80 function in the same pathway to stimulate DNA replication. BAP1 depletion did not affect the frequency of replication intermediates ( Fig. 5d,e ), indicating that, like INO80, BAP1 promotes fork progression rather than regulating replication initiation or termination. Consistently, BAP1 depletion reduced the average distance between replication origins ( Fig. 5f ). 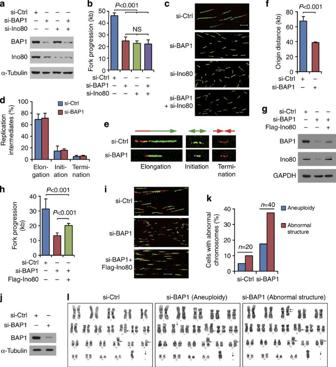Figure 5: BAP1 promotes replication fork progression via Ino80 stabilization and contributes to genome stability. (a) HeLa cells were transfected with BAP1- or Ino80-specific siRNAs or both, and then were subjected to immunoblotting. (b) The cells transfected as inawere subjected to the DNA fibre assay, and the results were graphed (n=3). NS, not significant. (c) Representative confocal images forb. (d) The frequency of the various replication intermediates ina–cwas graphed (n=3). (e) Representative confocal images ford. (f) The average origin distance ina–cwas graphed (n=3). (g) 293T cells transfected as indicated were subjected to immunoblotting. (h) The cells transfected as ingwere subjected to the DNA fibre assay, and the results were graphed (n=3). (i) Representative confocal images forh. (j) siRNA knockdown of BAP1 in HCT116 cells. (k) Karyotyping by mitotic spread. The percentages of the cells with aneuploidy or structural abnormalities were graphed (n=number of mitotic spreads). (l) Representative images fork. At least >300 fibres were counted for each sample in the DNA fibre assays shown. Error bars, mean±s.e.m. Figure 5: BAP1 promotes replication fork progression via Ino80 stabilization and contributes to genome stability. ( a ) HeLa cells were transfected with BAP1- or Ino80-specific siRNAs or both, and then were subjected to immunoblotting. ( b ) The cells transfected as in a were subjected to the DNA fibre assay, and the results were graphed ( n =3). NS, not significant. ( c ) Representative confocal images for b . ( d ) The frequency of the various replication intermediates in a – c was graphed ( n =3). ( e ) Representative confocal images for d . ( f ) The average origin distance in a – c was graphed ( n =3). ( g ) 293T cells transfected as indicated were subjected to immunoblotting. ( h ) The cells transfected as in g were subjected to the DNA fibre assay, and the results were graphed ( n =3). ( i ) Representative confocal images for h . ( j ) siRNA knockdown of BAP1 in HCT116 cells. ( k ) Karyotyping by mitotic spread. The percentages of the cells with aneuploidy or structural abnormalities were graphed ( n =number of mitotic spreads). ( l ) Representative images for k . At least >300 fibres were counted for each sample in the DNA fibre assays shown. Error bars, mean±s.e.m. Full size image To determine whether BAP1 exerts its activity for DNA replication by stabilizing Ino80, we ectopically expressed Ino80 in the cells depleted of BAP1. Although BAP1 depletion decreased Ino80 as shown previously, the ectopic expression of Ino80 in the BAP1-depleted cells elevated the Ino80 levels compatible to that of the control cells ( Fig. 5g ). Replication elongation was decreased by BAP1 depletion, as expected, which was only partially recovered by the elevation of Ino80 levels ( Fig. 5h,i ), indicating that BAP1 was still necessary for efficient fork progression although Ino80 was present at normal levels. These results suggest that BAP1 assists DNA replication not only by stabilizing Ino80 but also through other mechanisms. Our previous studies have shown that Ino80 deficiency causes numerical and structural abnormalities of chromosomes, a condition that was likely partly attributed to a replication defect [10] . Thus, we asked whether BAP1 deficiency would also lead to similar chromosomal defects. Indeed, depleting BAP1 from HCT116 cells increased both aneuploidy and structurally abnormal chromosomes ( Fig. 5j–l ), further confirming the agonistic role for BAP1 in the INO80-assisted DNA replication. These results are in agreement with a recent study showing that H226 cells lacking BAP1 exhibit severe chromosomal abnormalities under normal proliferation conditions [30] . BAP1 recruits INO80 to replication forks via H2Aub A recent study showed that BAP1 uses H2A monoubiquitinated at Lys-119 (H2Aub) in nucleosomes as a substrate and removes ubiquitin from H2A in vitro [31] . An earlier cytological study showed that H2Aub forms clusters partially co-localizing with PCNA foci in S phase [32] . These studies, together with our results thus far described, led us to investigate the possibility of a link between H2Aub and BAP1/INO80-assisted DNA replication. Overexpressing WT BAP1 in 293T cells, but not the C91S mutant, decreased H2Aub ( Fig. 6a ), and depleting BAP1 increased H2Aub ( Fig. 6b ), confirming that BAP1 uses H2Aub as a substrate within cells. Several studies have recently reported that BAP1 de-ubiquitinates H2Aub in human primary fibroblasts and U2OS osteosarcoma cells [30] , [33] , [34] , indicating that the cellular activity of BAP1 towards H2Aub is general. BAP1 interacted with H2Aub, and the ubiquitinating activity itself was not required for this interaction ( Fig. 6c ). As expected from BAP1 interacting with Ino80, Ino80 was associated with H2Aub in the cells ( Fig. 6d ). Notably, H2Aub formed clear nuclear foci overlapping with BAP1 and Ino80 in S-phase cells ( Fig. 6e ) and were found to associate with nearly all of the EdU-labelled chromatin fibres along with BAP1 and Ino80 ( Fig. 6f ). These data indicate that H2Aub, BAP1 and INO80 are all associated with replication forks for most of the time of DNA synthesis. 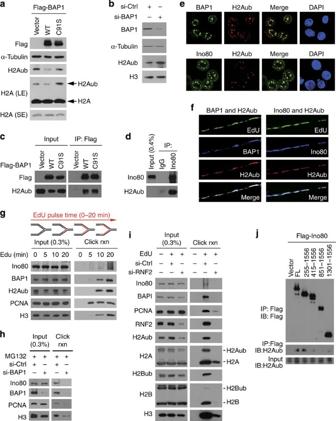Figure 6: BAP1 recruits INO80 to replication forks via the interaction with H2Aub. (a) After transfection with the WT or C91S Flag-BAP1 expression vectors, the cell lysates and acid extracts were prepared for immunoblotting analysis of the expression of Flag-BAP1 and histones, respectively. (b) The cells after transfection with siRNAs were subjected to immunoblotting as ina. (c) Flag-tagged proteins were immunoprecipitated from the cells expressing WT or C91S Flag-BAP1 and then were subjected to immunoblotting. (d) Immunoprecipitation for the interaction between Ino80 and H2Aub. (e) The cells were fixed and dually stained for BAP1 and H2Aub, and the confocal images of S-phase cells were captured. (f) Chromatin fibre assay. EdU-labelled, extended chromatin fibres were subjected to multiple staining for EdU, BAP1 and H2Aub (left) or for EdU, Ino80 and H2Aub (right). (g) iPOND assay. The cells were left untreated (0 h) or were treated with EdU for various times and then were processed according to the iPOND protocol. (h) The cells after transfection with siRNAs were treated with MG132 and processed according to the iPOND protocol after 20 min of EdU treatment. (i) The cells after transfection with siRNAs were left untreated or were treated with EdU for 20 min and then were processed according to the iPOND protocol. (j) After transfection with the indicated vectors, the cells were subjected to immunoprecipitation. 293T were used ina–dandj, and HeLa ine–i. Figure 6: BAP1 recruits INO80 to replication forks via the interaction with H2Aub. ( a ) After transfection with the WT or C91S Flag-BAP1 expression vectors, the cell lysates and acid extracts were prepared for immunoblotting analysis of the expression of Flag-BAP1 and histones, respectively. ( b ) The cells after transfection with siRNAs were subjected to immunoblotting as in a . ( c ) Flag-tagged proteins were immunoprecipitated from the cells expressing WT or C91S Flag-BAP1 and then were subjected to immunoblotting. ( d ) Immunoprecipitation for the interaction between Ino80 and H2Aub. ( e ) The cells were fixed and dually stained for BAP1 and H2Aub, and the confocal images of S-phase cells were captured. ( f ) Chromatin fibre assay. EdU-labelled, extended chromatin fibres were subjected to multiple staining for EdU, BAP1 and H2Aub (left) or for EdU, Ino80 and H2Aub (right). ( g ) iPOND assay. The cells were left untreated (0 h) or were treated with EdU for various times and then were processed according to the iPOND protocol. ( h ) The cells after transfection with siRNAs were treated with MG132 and processed according to the iPOND protocol after 20 min of EdU treatment. ( i ) The cells after transfection with siRNAs were left untreated or were treated with EdU for 20 min and then were processed according to the iPOND protocol. ( j ) After transfection with the indicated vectors, the cells were subjected to immunoprecipitation. 293T were used in a – d and j , and HeLa in e – i . Full size image The aforementioned results led us to hypothesize that BAP1 may recruit Ino80 to replication forks by interacting with H2Aub. To test this hypothesis, we employed the recently developed technology called isolation of proteins on nascent DNA (iPOND), which involves EdU labelling of replicating DNA and covalent linkage to a biotin-azide by click reaction to facilitate single-step purification of the EdU-labelled nascent DNA with associated proteins for the detection of the proteins bound at active replication forks [35] , [36] . PCNA and histone H3 were detected on the chromatin purified from the EdU-treated cells with their levels proportionally increasing to the click reaction time, whereas they were not detected from the samples of untreated cells ( Supplementary Fig. 4 ), validating the assay. Using this assay, we were able to confirm the association of Ino80, BAP1 and H2Aub with replication forks ( Fig. 6g ). We then asked whether BAP1 is required for Ino80 recruitment to replication forks. The Ino80 recruitment to replication forks was abolished upon BAP1 depletion in the cells treated with MG132 (to prevent Ino80 degradation caused by BAP1 depletion; Fig. 6h ), indicating that Ino80 could not bind to replication forks in the absence of BAP1. As a result, DNA replication was severely compromised as evidenced by a large decrease of the fork-associated PCNA and H3 ( Fig. 6h ). Next, we determined whether Ino80 recruitment to replication forks is mediated by interaction between BAP1 and H2Aub. RNF2 (also called Ring1b or Ring2), the major H2A ubiquitin ligase [37] , was associated with replication forks as expected. On RNF2 depletion, RNF2 and H2Aub were not detected at replication forks. Notably, BAP1 and Ino80 were no longer recruited to the replication forks. Consistently, DNA replication was severely compromised on RNF2 depletion as manifested by a large decrease of the fork-associated H3 and PCNA ( Fig. 6i ). Consistently, the Ino80 mutant lacking the HSA domain important for the interaction with BAP1 failed to associate with H2Aub ( Fig. 6j ). Furthermore, BAP1 depletion compromised the formation of Ino80 foci in S-phase cells ( Supplementary Fig. 5 ). Taken together, these results suggest that BAP1 recruits INO80 to replication forks based on the interaction with H2Aub. These findings explain why restoring the Ino80 levels by ectopic expression only partially rescued the replication defects in BAP1-depleted cells. A recent study reported that H2B monoubiquitination at Lys-120 (H2Bub) has an important role in fork progression and replisome stability in yeast [38] . Interestingly, we observed that H2Bub was also associated with replication forks ( Fig. 6i ). Confirming this result, H2Bub formed the nuclear foci overlapping with BAP1 and Ino80 in S phase ( Supplementary Fig. 6a ) and associated with EdU-labelled chromatin in much the same way as H2Aub ( Supplementary Fig. 6b ). Therefore, we examined a potential role for H2Bub in INO80 recruitment and/or DNA replication. Depleting RNF20, the major H2B ubiquitin ligase [39] , [40] , largely deprived replication forks of H2Bub. However, the RNF20 depletion neither affected the recruitments of BAP1 and Ino80 to replication forks nor compromised replication fork progression ( Supplementary Fig. 6c ). Thus, unlike in yeast, H2Bub may have other roles than fork progression in DNA replication in human cells. Ino80 is downregulated in BAP1-defective mesothelioma Given that BAP1 is deleted or inactivated in various human cancers, we investigated the possibility that Ino80 is downregulated in BAP1 -defective cancer cells. First, we compared the Ino80 levels between MSTO-211H and H226 cells, the MPM lines normally expressing BAP1 and lacking BAP1 expression, respectively. MSTO-211H expressed BAP1 at the compatible levels of 293T cells, whereas H226 showed no BAP1 expression ( Fig. 7a ). Strikingly, the Ino80 levels in H226 cells were very low compared with those in MSTO-211H cells and was recovered to a large extent by BAP1 expression ( Fig. 7b ). The Ino80 levels in H226 cells achieved by BAP1 expression were even higher than those obtained by an ectopic overexpression of Ino80 ( Fig. 7b ). The recovery of Ino80 in H226 cells required the catalytic activity and Ino80-interacting domain of BAP1 ( Fig. 7c ), indicating that the Ino80 recovery by BAP1 was specific. Importantly, the Ino80 levels in H226 cells also could be recovered by MG132 treatment ( Fig. 7c ). These results show that the Ino80 decrease in H226 cells was specifically due to the lack of BAP1, which would otherwise have maintained Ino80 at normal levels by preventing proteasomal degradation. 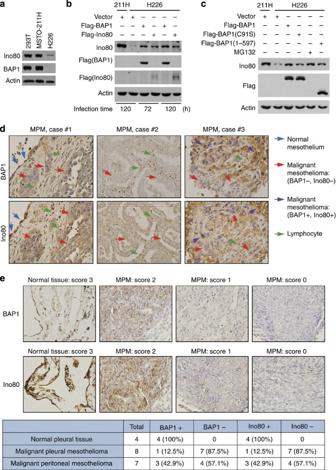Figure 7: Ino80 is downregulated in BAP1-defective mesothelioma. (a) Immunoblot analysis for Ino80 and BAP1 expression in the indicated cells. (b) The cells were infected with empty vector, or Flag-BAP1- or Flag-Ino80-expressing (as control) lentiviruses for 72 or 120 h, and lysates were subjected to immunoblotting. (c) The cells were infected with the indicated lentiviruses for 120 h or treated with MG132 before being subjected to immunoblotting. (d) Immunohistochemistry for BAP1 and Ino80 expression in the paraffin-embedded frozen tumours from three MPM patients (Seoul National University Hospital). (e) Immunohistochemical staining of BAP1 and Ino80 in normal mesothelial tissues, malignant pleural and peritoneal mesothelioma using tissue microarray (US Biomax, MS801). The results of the scoring of BAP1 and Ino80 expression are shown in the lower table. Figure 7: Ino80 is downregulated in BAP1-defective mesothelioma. ( a ) Immunoblot analysis for Ino80 and BAP1 expression in the indicated cells. ( b ) The cells were infected with empty vector, or Flag-BAP1- or Flag-Ino80-expressing (as control) lentiviruses for 72 or 120 h, and lysates were subjected to immunoblotting. ( c ) The cells were infected with the indicated lentiviruses for 120 h or treated with MG132 before being subjected to immunoblotting. ( d ) Immunohistochemistry for BAP1 and Ino80 expression in the paraffin-embedded frozen tumours from three MPM patients (Seoul National University Hospital). ( e ) Immunohistochemical staining of BAP1 and Ino80 in normal mesothelial tissues, malignant pleural and peritoneal mesothelioma using tissue microarray (US Biomax, MS801). The results of the scoring of BAP1 and Ino80 expression are shown in the lower table. Full size image Next, we analysed the expression of BAP1 and Ino80 in tumour tissues from three MPM patients by immunohistochemistry. We validated the antibodies against BAP1 and Ino80 for immunohistochemistry using paraffin-embedded frozen tissues ( Supplementary Fig. 7 ). In tumours from the first two cases, both BAP1 and Ino80 were stained weakly in mesothelioma cells but strongly in mesothelial cells ( Fig. 7d ). The tumour from the last case showed mesothelioma cells with either strong or weak staining of both BAP1 and Ino80 ( Fig. 7d ). These data support a correlation between BAP1 and Ino80 expression in mesothelioma cells of MPM tumours. Furthermore, we analysed the expression of BAP1 and Ino80 in mesothelioma using tissue microarrays. We scored the staining of BAP1 and Ino80 each from 0 to 3 and arbitrarily designated scores 0–1 as negative and scores 2–3 as positive. Although all of the four normal pleural tissues analysed were scored as BAP1 positive, seven of eight MPM (87%) and four of seven malignant peritoneal mesothelioma tissues (57%) were scored as BAP1 negative, showing a high frequency of BAP1 defects in these tumours. Notably, all of the tumours scored as BAP1 negative were scored as Ino80 negative, and all of the normal and tumour tissues scored as BAP1 positive were scored as Ino80 positive ( Fig. 7e and Supplementary Fig. 8 ). These results show a strong positive correlation between BAP1 and Ino80 expression in mesothelioma cells. In the present study, we demonstrated that INO80 promotes replication fork progression during normal DNA synthesis. We also found that the cellular level of Ino80 is regulated by the ubiquitin–proteasome pathway, and BAP1 stabilizes Ino80 by de-ubiquitination. Importantly, BAP1 recruits INO80 to replication forks through the interaction with H2Aub to promote fork progression. Consistent with its roles in Ino80 stability and DNA replication, BAP1 is required for genome integrity during normal cell proliferation. INO80 may increase DNA accessibility by disrupting or mobilizing nucleosomes ahead of the fork to facilitate DNA unwinding and polymerase movement. Alternatively, but not exclusively, INO80 could function to assemble nucleosomes and restore pre-replication chromatin behind the fork, a process that is also thought to be important for efficient fork progression ( Fig. 8 ). 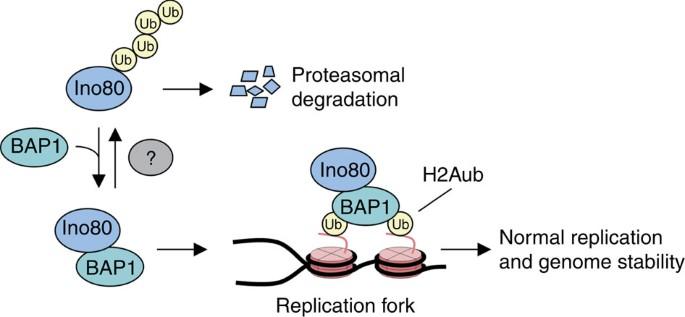Figure 8: Model for the role of BAP1 and INO80 in DNA replication. The stability of Ino80 is regulated by the opposing activities of BAP1 and yet-to-be identified Ino80 ubiquitin ligase. In normal cells, BAP1 stabilizes by de-ubiquitination and recruits Ino80 to replication forks based on the interaction with H2Aub, ensuring efficient fork progression and genome stability. In BAP1-null cells, such as H226 cells, Ino80 undergoes proteasomal degradation via ubiquitination and fails to associate with replication forks, leading to defective replication and genome instability. Only Ino80 of the INO80 complex is shown for clarity. Figure 8: Model for the role of BAP1 and INO80 in DNA replication. The stability of Ino80 is regulated by the opposing activities of BAP1 and yet-to-be identified Ino80 ubiquitin ligase. In normal cells, BAP1 stabilizes by de-ubiquitination and recruits Ino80 to replication forks based on the interaction with H2Aub, ensuring efficient fork progression and genome stability. In BAP1-null cells, such as H226 cells, Ino80 undergoes proteasomal degradation via ubiquitination and fails to associate with replication forks, leading to defective replication and genome instability. Only Ino80 of the INO80 complex is shown for clarity. Full size image Although a previous cytological study found that Ino80 foci colocalized with PCNA [10] , that study could not determine whether Ino80 binds to replication forks due to the limitation of the microscopic resolution. Thus, there was no direct evidence for the involvement of INO80 in DNA replication. In the current study, we showed Ino80 binding to replication forks at the single DNA molecule level using immunofluorescence and at the whole molecule level using highly sensitive biochemical methodology. These results, together with the observations that Ino80 depletion severely compromises replication fork progression, strongly support the direct role of INO80 in this process. However, because INO80 regulates the transcription of many cellular genes, the possibility cannot be formally excluded that INO80 also contributes to replication fork progression via gene expression. DNA replication is the key process for cell division and proliferation. Thus, the role of INO80 in DNA replication likely accounts, to a large extent, albeit not fully, for the early embryonic lethality of Ino80 -null mice. Very recently, a conditional gene-targeting study in mice reported similar results as ours that Ino80 disruption results in early embryonic lethality [41] . That study also showed that Ino80 -null MEFs are defective in S-phase progression and BrdU incorporation, consistent with our conclusion for the Ino80 role in normal DNA replication. It has been reported that BRG1, the catalytic subunit of mammalian SWI/SNF complexes, participates in replication fork progression in mouse embryos and human fibroblasts, highlighting the conserved role for the SWI/SNF family chromatin-remodelling complexes in DNA replication [42] . Does INO80 function in mammalian DNA replication under stressed conditions as it does in yeast? A study in mice showed that Ino80 disruption resulted in increased fragility of telomeres (thereby accelerating defective telomere replication) [41] , resembling the common fragile sites that are specific genomic regions prone to break under replication stress. A recent genome-wide profiling study showed that, upon increased replication stress by activated cell proliferation, Ino80 is colocalized with the histone H2AX that is dynamically reorganized to preoccupy the hotspots of γ-H2AX (phosphorylated H2AX), the DNA double-strand break marker found at stalled replication forks [43] . These results raised a possibility that mammalian INO80 has roles in the recovery of stalled replication forks and repair of replication stress-induced DNA damage. Indeed, we have observed that the Ino80 level increased when HeLa cells were treated with HU (H.-S.L. and J.K., unpublished observations). However, the role of mammalian INO80 in stressed replication and damage tolerance remains to be investigated. Although yeast INO80 has been shown to associate with origins of replication and stalled replication forks, the mechanisms responsible for INO80 recruitment remain unknown. INO80 is recruited to the sites of DNA double-strand breaks by direct interaction with γ-H2AX in yeast [44] , [45] , and recruitment of the SMARCAD1and SNF2H chromatin remodelers to replication forks is mediated by PCNA in human cells [46] , [47] . In this regard, involvement of BAP1 in INO80 recruitment to replication forks is unexpected and novel. However, the mechanisms by which BAP1 recruits INO80 to replication forks remain to be elucidated. Although our data suggest that H2Aub is important for this process, other factors such as histone markers other than H2Aub and replication proteins also likely have a role. Interestingly, while the Ino80 subunit is conserved between yeast and humans, Yuh1, the unique BAP1 ortholog in yeast, lacks the C-terminal extension containing the BRCA1 interaction domain that is critical for the interaction with Ino80 (ref. 48 ), suggesting that the mechanism for the BAP1-mediated INO80 recruitment does not likely exist in yeast. Therefore, it seems that the mechanisms to recruit chromatin remodelers to replication forks are not only remodeler-type specific but also evolutionarily diversified. The Ino80-stabilizing activity of BAP1 should not necessarily be specific to DNA replication but will likely affect INO80 functions in general. Indeed, that BAP1 interacts with Ino80 throughout the cell cycle with the Ino80 level remaining unchanged suggests a constitutive role for BAP1 in INO80 functions. Although this could be the case at least for normally cycling cells, BAP1 may regulate Ino80 stability by responding to certain physiological conditions, such as DNA damage and replication stress. Interestingly, BAP1 is phosphorylated in response to various agents that induce DNA damage and replication stress, including HU [30] , [49] . It will be interesting to investigate the potential impact of this BAP1 modification on the increase of Ino80 after HU treatment. In keeping with our finding of BAP1 activity in the regulation of Ino80, it has recently been reported that the ubiquitin-conjugating enzyme UBE2O sequesters BAP1 in the cytoplasm by ubiquitinating its nuclear localization signal, resulting in an increase in Ino80 ubiquitination and a decrease in the Ino80 level [50] . If H2Aub at replication forks functions in INO80 recruitment, why do BAP1 and RNF2 have opposing activities on H2Aub recruited to the forks? The ubiquitin ligases for H2Aub are associated with transcriptional repressive complexes, and H2Aub is thought to function as a repressive marker for transcription possibly by regulating higher order chromatin structure. Polycomb repressive complex 1 (PRC1), one of the main families of Polycomb group protein complexes, contains RNF2 and silences target gene expression [51] . In Drosophila , repression of Polycomb group target genes requires the H2A ubiquitinase activity of PRC1 as well as the de-ubiquitinase activity of Polycomb repressive de-ubiquitinase, a complex comprising Calypso ( Drosophila homologue of BAP1) and ASX [31] . Although this observation seems paradoxical, it has been suggested that Polycomb repressive de-ubiquitinase may help to fine-tune gene expression levels by preventing hyperubiquitination by PRC1. By analogy with this mechanism, both BAP1 and RNF2 activities may be needed to make fine adjustments to H2Aub levels for optimal chromatin compactness ahead of a replication fork and/or on newly replicated DNA during fork progression. The ability of BAP1 to suppress cell growth (for example, H226 cell growth) could account for its tumour suppressor function. However, several studies have reported that BAP1 also promotes cell proliferation. For example, BAP1 depletion decreases the growth of various human cells, including BAP1-expressing mesothelioma lines such as HMeso and MSTO-211H (refs 18 , 52 ). In contrast to the case of H226 cells, re-expression of BAP1 modestly increases the proliferation of other types of BAP1-null mesothelioma cells, such as Meso37 and H28 (ref. 18 ). Although BAP1 can promote cell proliferation by accelerating G1/S progression via host cell factor-1 activation [52] , [53] , our results suggest that BAP1 can also contribute to cell proliferation by promoting replication fork progression. Indeed, BAP1 depletion results in an accumulation of cells in S phase; conversely, BAP1 re-expression in BAP1-null cells reduces cells in S phase [18] , [53] , [54] . Thus, the impact of BAP1 on cell proliferation appears to manifest as the combined effects on DNA replication and other cellular pathways that control cell cycle progression. Although BAP1 activity to stimulate replication and cell proliferation seems paradoxical for its tumour suppressor function, we speculate that its activity to suppress genome instability may be more important. In summary, we have established the role of INO80 in normal DNA replication and have found that BAP1 has a dual function in regulating INO80 activity in the replication process: INO80 stabilization and recruitment of INO80 to replication forks. These results reveal an unexpected mechanism that targets INO80 to replication forks and provide a novel insight into the molecular basis for the BAP1 tumour suppressor function by linking this protein to genome replication and stability. Highlighting the clinical significance of our findings, Ino80 is downregulated in BAP1-defective mesothelioma likely due to the lack of the Ino80 stabilization mechanism of BAP1, implying that inactivating mutations of BAP1 can cause Ino80 downregulation during tumorigenesis. Given the critical role for INO80 in genome stability, it is tempting to hypothesize that BAP1 contributes to tumour suppression through the mechanism of Ino80 stabilization. It will be of great interest to investigate whether and to what extent the tumorigenic capacity of BAP1-null cancer cells, such as H226 cells, can be diminished by Ino80 expression. Cells and antibodies MSTO-211H and H226 cells were purchased from ATCC and were maintained in RPMI-1640 supplemented with 10% fetal bovine serum (FBS). The sources and optimal working dilutions of the antibodies used in the study are summarized in Supplementary Table 2 . Uncropped western blots are shown in Supplementary Fig. 9 . Plasmids, siRNA and transfection The plasmid vectors expressing full-length and truncated Flag-Ino80, as well as full-length Myc-Ino80, have been described previously [10] , [55] , [56] . The expression vectors for Flag-BAP1, Flag-BAP1(1–597) and Flag-BAP1(598–729) were generated by cloning the corresponding sequences that were amplified by PCR from the human BAP1 cDNA into p3XFlag-CMV-14 vector (Sigma). The vector expressing Flag-BAP1(C91S) was generated by site-directed mutagenesis according to the QuickChange mutagenesis protocol using Pfu turbo polymerase (Stratagene). The expression vectors for Myc-BAP1 and Myc-BAP1(C91S) were generated by cloning the full-length BAP1 sequences that were amplified by PCR from Flag-BAP1 and Flag-BAP1(C91S), respectively, into pcDNA3.1/myc-his(-). The lentiviral vectors expressing Flag-BAP1, Flag-BAP1(C91S) or Flag-Ino80 were generated by cloning the corresponding cDNA sequences into the pCDH-CMV-MCS-EF1-copGFP vector (System Biosciences). All of the newly constructed plasmid vectors were verified by sequencing. The detailed procedures for vector construction and the sequence information for the oligonucleotides used are available upon request. The sequences of siRNA used were as follows: si-Ino80, 5′- uuaagagugugauuucucauu and 5′- ugagaaaucacacucuuaauu ; si-control, 5′- ccuacgccaccaauuucguuu and 5′- acgaaauugguggcguagguu ; si-BAP1, 5′- cuccaucagaccaauccaa and 3′- uuggauuggucugauggag ; si-RNF2, 5′- ccuaguaacaaacggacca (dTdT) and 5′- ugguccguuucuuacuagg (dTdT); and si-RNF20, 5′- cugcacgggccuuggaaa and 5′- uuuuccaaggcccgugcag . Transfections of plasmids and synthetic siRNA were performed using the calcium phosphate method or Lipofectamine 2000 (Invitrogen) typically for 48 h. DNA fibre assay The DNA fibre assay was performed essentially as previously described [28] . The cells were treated sequentially with IdU for 10 min and CldU for 30 min each at 100 μM, collected by trypsinization and resuspended in phosphate-buffered saline (PBS). Approximately 400 cells were plated on a Silane-Prep Slide (Sigma-Aldrich; S4651) and air dried for 7 min; next, 10 μl of the spreading buffer (0.5% sodium dodecyl sulphate (SDS), 200 mM Tris-Cl (pH 7.4), 50 mM EDTA) was added. After 10 min of incubation, the slides were tilted slowly for 2 h to extend the DNA fibres. After fixation with 3:1 methanol/acetic acid for 2 min, the cells on the slides were washed twice with PBS and stored overnight at −20 °C. The slides were treated with 2.5 N HCl for 30 min to denature the extended DNA fibres and washed twice with PBS followed by incubation in 2% bovine serum albumin (BSA) for 40 min. The slides were incubated with a mixture of mouse anti-BrdU (for IdU detection) and rat anti-BrdU (for CldU detection) at room temperature (RT) for 1 h and then were incubated with stringency buffer (10 mM Tris-Cl (pH 7.4), 400 mM NaCl, 0.2% Tween-20, 0.2% NP-40) at RT for 10 min to remove nonspecific binding. After washing three times with PBS, the slides were incubated with a mixture of secondary antibodies (Alexa Fluor 568 rabbit anti-mouse IgG (Invitrogen; A11061) and Alexa Fluor 488 chicken anti-rat IgG (Invitrogen; A21470)) at RT for 30 min and then with another mixture of secondary antibodies (Alexa Fluor 568 goat anti-rabbit IgG (Invitrogen; A11011) and Alexa Fluor 488 goat anti-chicken IgG (Invitrogen; A11039)) after 15 min of blocking. After washing three times with PBS, the slides were mounted using Vectashield mounting medium. All fluorescence microscopic images were generated using a Carl Zeiss LSM510 scanning laser confocal microscope. The average track lengths of fork progression were calculated by considering only DNA fibres representing ongoing forks (total length of red-green tracks) and converting to base pairs on the basis of 1-μm-long DNA being equivalent to approximately 2.8 kb. Chromatin fibre assay The chromatin fibre assay was performed as previously described with minor modifications [27] . Briefly, the cells were treated with 10 μM EdU (Invitrogen) for 30 min, collected by trypsinization and resuspended in 75 mM KCl followed by incubation at 37 °C for 30 min. The cells were plated on Superfrost Plus Slides (Fisher Scientific) and air dried for 10 min; next, lysis buffer (25 mM Tris-Cl pH 7.5, 0.5 M NaCl, 1% Triton X-100, 0.2 M urea) was added. After incubation at RT for 10 min, the cells were covered with a coverslip and air dried overnight. After the coverslips were removed, the slides were incubated with potassium chromosome medium (KCM) buffer (120 mM KCl, 20 mM NaCl, 10 mM Tris-Cl (pH 7.5), 0.5 mM EDTA, 0.1% (v/v) Triton X-100) at RT for 30 min and blocked with 10% BSA/KCM for 30 min. The slides were incubated with primary antibodies for 1 h, washed with KCM buffer, incubated with secondary antibodies for 30 min and then rinsed three times with KCM buffer. To fix chromatin fibres, the slides were incubated with 4% formaldehyde in KCM buffer and then washed with KCM buffer for 5 min. The slides containing EdU-labelled chromatin fibres were incubated with Click-iT EdU Alexa Fluor 488 Imaging Kit solution for 30 min, washed three times with KCM buffer and mounted by Vectashield before confocal images were captured using a Carl Zeiss LSM510 microscope. Generation of Ino80 knockout mice The Ino80 targeting vector was generated by cloning the 2543-bp Not1-Sal1 genomic fragment containing intron 1 and the 7263-bp BamH1-Kpn1 genomic fragment containing exons 5, 6 and 7 into the PGK-neo gene in the pPNT vector as left and right arms, respectively. The target vector was transfected into ES cells from the 129/Sv strain, and the targeted ES cells were screened and injected into blastocysts from the C57BL/6 strain. The resulting blastocysts were implanted into a C57BL/6 surrogate mother, and chimeric mice were obtained. The chimeric mice were bred with normal C57BL/6 mice, and the first Ino80 heterozygous agouti male mouse was obtained. To generate Ino80 +/ − mice congenic to C57BL/6, the founding Ino80 +/ − agouti male mouse was crossed with a C57BL/6 female, and the resulting Ino80 +/ − mice (N1) were repeatedly backcrossed to C57BL/6 mice until N7 mice were obtained. All of the animal experiments in the current study were performed in compliance with the ethical guidelines of the Institutional Animal Care and Use Committee of Ewha Womans University. Southern blot analysis Genomic DNA was extracted by digesting tail biopsies in lysis buffer (50 mM Tris-Cl (pH 8.0), 100 mM EDTA (pH 8.0), 100 mM NaCl, 1% SDS and 600 μg ml −1 proteinase K) at 55 °C for 12–16 h, followed by precipitation with NaCl and 70% cold ethanol. After washing with 100% ethanol, the DNA was dissolved in sterile water and stored at 4 °C until use. Genomic DNA (15 μg) was digested with EcoRV at 37 °C for 16–20 h and separated on a 0.8% agarose gel in TAE at 25 V at 4 °C for 16 h. After treatment with denaturing solution (0.5 N NaOH, 1.5 M NaCl) for 30 min, the DNA was neutralized and transferred to Hybond N+ nylon membrane (GE Healthcare) for 16–20 h using an alkaline buffer (0.3 M Na 3 citrate, 3 M NaCl). The membrane was cross linked with UV and pre-hybridized with hybridization solution (Millipore) at 42 °C for 3–4 h. Next the membrane was hybridized at 42 °C for 16–20 h using the 460-bp DNA probe that was amplified by PCR from the mouse genomic DNA using the oligonucleotides 5′- gggctgtgttgtggttctaaggag and 5′- taccaccccttatctatgggtctc and labelled with [α- 32 P]-dCTP by random-primed DNA synthesis (Roche). After three washes with 2 × SSC with 0.5% SDS at 65 °C for 20 min to remove nonspecific binding, the membrane was exposed to X-ray film at −80 °C overnight. PCR genotyping Genomic DNA was extracted from mouse tails and embryos using lysis buffer (50 μg ml −1 proteinase K, 50 mM Tris-Cl (pH 8.0), 1% SDS, 100 mM EDTA (pH 8.0) and 100 mM NaCl) and Direct PCR lysis buffer (VIAGEN), respectively. Genotyping was performed by PCR using primers 1 and 2 for the WT allele (430-bp product) and primers 1 and 3 for the targeted allele (280-bp product). The primer sequences were as follows: primer 1, 5′- gtggaggacaaataggaagtgag -3′; primer 2, 5′- gaaatattcctgttgaagatggct g -3′; primer 3, 5′- ccagaggccacttgtgtagcgccaag -3′. Preparation and maintenance of MEF cells Embryos were isolated from mothers at 3.5 days post conception (d.p.c.) and were subjected to MEF preparation. MEFs were cultured in medium (DMEM supplemented with 10% FBS, 10,000 U ml −1 antibiotic–antimycotic solution) according to the 3T9 schedule; cells were plated at 9 × 10 5 per 10-mm dish and were passaged at 3-day intervals. In vitro culture of mouse embryos In vitro culture of mouse embryos was performed according to the standard protocols (Manipulating the mouse embryo: A laboratory manual. 2003, 3rd Edition, New York: Cold Spring Harbor Laboratory Press). Two-cell embryos were isolated from 1.5-d.p.c. pregnant mothers by flushing the uterus with M2 media (Sigma-Aldrich). Isolated embryos were cultured for 3 days in a droplet of M16 media (Sigma-Aldrich) embedded in mineral oil (Sigma-Aldrich) to allow the embryos to develop into blastocysts, which were further cultured for 4 days in a droplet of the ES cell medium (DMEM supplemented with 15% FBS, 2 mM L-glutamine, 0.1 mM MEM non-essential amino acids, 50 μg ml −1 pen per strep, 0.1 mM 2-mercaptoethanol, 1,000 units ml −1 mouse LIF) embedded in mineral oil. For blastocyst culture, embryos were isolated from 3.5-d.p.c. mothers and cultured for 1 day in a droplet of the M16 medium embedded in mineral oil to allow for blastocyst expansion, followed by further culturing in the ES cell medium for up to 6 days. DNA fibre assay for mouse embryos The embryos isolated from pregnant mothers at 3.5-d.p.c. were cultured for 1 day in a droplet of the M16 medium embedded in mineral oil, and sequentially treated with IdU for 10 min and CldU for 30 min each at 100 μM. To remove the zona pellucida, the embryos were treated with acid Tyrode’s solution for a few seconds and washed several times with PBS. The embryos were then placed on a Silane-Prep Slide and subsequently processed as described in the assay for cultured cells. Yeast two-hybrid screen The yeast two-hybrid screen was performed using the Matchmaker GAL4 Two Hybrid System 3 (Clontech). The sequences corresponding to the three subdomains of human Ino80 (the amino (N)-terminal region containing the HSA domain, aa 1–500; the central region containing the ATPase domain, aa 501–1,300; the C-terminal region, aa 1,301–1,556) were amplified by PCR from the pcDNA-hINO80 vector and cloned into the bait plasmid vector pGBKT7. The sequences of the PCR primers used were as follows: the N-terminal region, 5′- gaattcagacagatttgttctatggcctcggagttg -3′ and 5′- gctggtcgacataactctccccaaacccagtgccagactt -3′; the central region, 5′- cgaattcagcctggctaacccatctat -3′ and 5′- gctggtcgactttcactcggttggtttc -3′; the C-terminal region, 5′- cgaattcgagcgcaagcggaagcggga -3′ and 5′- gctggtcgacttaccgtcctccagaggg -3′. Screening was conducted according to the manufacturer's protocols using the AH109 strain after transformation with the Human Prostate Matchmaker cDNA library. Positive colonies were selected under high-stringency conditions on SD/-Ade/-His/-Leu/-Trp plates. The selected positive colonies were confirmed by the colony-lift filter assay (β-Galactosidase assay). iPOND assay The iPOND assay was conducted according to the procedure described previously [36] . The cells were fixed with 1% formaldehyde for 20 min at RT following a pulse with 10 μM EdU, and 0.125 M glycine was added to stop the fixing reaction. After washing three times with PBS, the cells were resuspended in 0.25% Triton X/PBS and incubated for 20 min for permeabilization. The cells were then washed sequentially with 0.5% BSA/PBS and PBS, and incubated in the Click-iT Cell Reaction Buffer Kit (Invitrogen) containing 1 mM biotin-azide for 2 h in the dark. After a sequential wash as described before, the cells were lysed by incubation with lysis buffer (1% SDS, 50 mM Tris-Cl (pH 8.0), protease inhibitor cocktail) for 30 min on ice and subjected to sonication at a 30% amplitude setting using a Cole-Parmer 400 Watt Ultrasonic Homogenizer (three times, 10 s each). The cell lysates were centrifuged at 8,000 g for 10 min, and the supernatant was filtered through a 100-μm nylon mesh followed by the addition of the same volume of PBS. The resulting supernatant was incubated with Streptavidin-agarose beads (Novagen) overnight at 4 °C and centrifuged as described above. After washing three times with the lysis buffer, the pellet was suspended in SDS sample loading buffer and boiled for 25 min before being subjected to SDS–PAGE and immunoblot analysis. Immunohistochemistry The cultured cells were fixed with methanol for 10 min (4% formaldehyde for 20 min for Ino80 staining) at RT, permeablized by incubating in 0.2% Triton X/PBS for 10 min and blocked by treating with 1% BSA for 1 h. After four washes with PBS (10 min each), cells were incubated with primary antibodies overnight at 4 °C, and incubated with Alexa Fluor-conjugated antibodies (Molecular Probes) after washing as described above. After washing, cells were mounted using Vectashield mounting medium with 4′,6-diamidino-2-phenylindole (DAPI; Vector Laboratories) before confocal images were captured using a Carl Zeiss LSM510 microscope. The 3-μm-thick paraffin-embedded frozen tissue sections mounted on slides were deparaffinized in xylene and rehydrated using decreasing concentrations of ethanol. The tissue sections were incubated in sodium citrate buffer (10 mM sodium citrate, 0.05% Tween-20 (pH 6.0)) at 95 °C for 30 min for antigen retrieval and then were treated with 3% hydrogen peroxide for 5 min to block endogenous peroxidase activity. For blocking, the slides were incubated in PBS with 1% BSA at RT for 1 h. Primary antibodies diluted in 1% blocking serum (anti-BAP1 antibody, 1:100; anti-Ino80 antibody, 1:400) were added onto the tissue sections followed by overnight incubation at 4 °C. After several washes, the tissue sections were sequentially incubated with pre-diluted biotinylated goat anti-rabbit IgG for 1 h and with VECTASTAIN ABC Reagent (Vector Laboratories). Immunoreactive cells were visualized by the addition of DAB chromogen (Vector Laboratories) and a haematoxylin counterstain before images were taken using an Olympus BX 51 light microscope. Informed consent was obtained for the experiments with the tumour tissues from MPM patients at Seoul National University Hospital. Immunoprecipitation The cells were lysed in NETN buffer (20 mM Tris-Cl (pH 8.0), 150 mM NaCl, 1 mM EDTA (pH 8.0), 0.5% NP-40, 0.1 mM phenylmethylsulphonyl fluoride and protease inhibitor cocktail) on ice for 30 min and subjected to sonication at 30% amplitude using a Cole-Parmer Ultrasonic Homogenizer (three times, 10 s each). After clarification by centrifugation at 12,000 rpm at 4 °C for 10 min, the lysates were pre-cleared by incubating with protein G Sepharose at 4 °C for 2 h followed by centrifugation. The resulting supernatants were incubated with primary antibodies overnight and further incubated with protein G Sepharose for 3 h. After washing several times with NETN buffer, the pellet was suspended in SDS sample loading buffer and boiled for 5 min before being subjected to SDS–PAGE and immunoblot analysis. Lentivirus infection The lentiviral vectors were transfected into HEK-293T cells using the FuGENE HD transfection reagent (Promega). After 48 h, the virus-containing medium was harvested, filtered through a 0.45-μm syringe filter to remove residual cells and used for target cell infection. Statistical analysis The significance of differences between measurements was evaluated by Student’s t -test using Microsoft Excel. A P value <0.05 was deemed to indicate statistical significance. How to cite this article: Lee, H.-S. et al . Stabilization and targeting of INO80 to replication forks by BAP1 during normal DNA synthesis. Nat. Commun. 6:5128 doi: 10.1038/ncomms6128 (2014).